The origin of pelletal lapilli in explosive kimberlite eruptions Kimberlites are volatile-rich magmas from mantle depths of ≥150 km and are the primary source of diamonds. Kimberlite volcanism involves the formation of diverging pipes or diatremes, which are the locus of high-intensity explosive eruptions. A conspicuous and previously enigmatic feature of diatreme fills are 'pelletal lapilli'—well-rounded clasts consisting of an inner 'seed' particle with a complex rim, thought to represent quenched juvenile melt. Here we show that these coincide with a transition from magmatic to pyroclastic behaviour, thus offering fundamental insights into eruption dynamics and constraints on vent conditions. We propose that pelletal lapilli are formed when fluid melts intrude into earlier volcaniclastic infill close to the diatreme root zone. Intensive degassing produces a gas jet in which locally scavenged particles are simultaneously fluidised and coated by a spray of low-viscosity melt. A similar origin may apply to pelletal lapilli in other alkaline volcanic rocks, including carbonatites, kamafugites and melilitites. Kimberlite melts ascend from the Earth's mantle to the surface in a matter of hours to days [1] , [2] . Their diatreme-hosted deposits provide valuable insights into the dynamics of other volcanic conduits and represent the main source of diamonds on Earth. Kimberlite diatremes are subject to a wide range of volcanic and sedimentary processes and interactions [3] , [4] , and in some cases, are host to exceptional fossil preservation [5] . Additionally, the xenoliths and xenocrysts they contain provide valuable information on the structure and composition of the deep subcontinental mantle [6] , [7] . Most volcaniclastic kimberlites contain ubiquitous yet poorly understood composite particles termed 'pelletal lapilli' [1] , [8] , [9] , [10] , [11] , [12] . These are defined as discrete sub-spherical clasts with a central fragment, mantled by a rim of probable juvenile origin [9] . Pelletal lapilli typically range in size from <1–60 mm, and occur both as accessory components of pipe-filling volcaniclastic kimberlites and as the main pyroclast type in narrow, steep-sided 'pipes' within the diatreme. These clasts have previously been attributed to incorporation of particles into liquid spheres in the rising magma [8] , [13] and rapid unmixing of immiscible liquids [14] . However, these models fail to explain many aspects of their internal structure, composition and abundance in pyroclastic intrusions. Pelletal lapilli have been identified globally in a wide range of other alkaline volcanic rocks, including carbonatites [15] , kamafugites [13] , [16] , melilitites [14] , [15] and orangeites [17] . They have also been referred to as 'tuffisitic lapilli' [15] , 'spherical lapilli' [18] , 'spinning droplets' [13] , [19] and 'cored lapilli' [20] , [21] . Although pelletal lapilli are similar in appearance and structure to 'armoured' (or cored) lapilli [22] , the latter are formed by accretion of moist fine-grained ash (as opposed to liquid melt) to the central fragment [23] , [24] . Pelletal lapilli share similar properties to particles formed during industrial fluidised granulation processes, but such processes have not previously been considered in a geological context. Fluidised spray granulation is widely used in industrial engineering to generate coated granules with specific size, density and physicochemical properties [25] , [26] . The mechanism involves continuous injection of atomisable liquids, solutions or melts into a powdery fluidised bed [27] , which produces a dispersion of larger coated granules that are simultaneously dried by the hot fluidising gas [27] , [28] . When gas flows upwards through particles, the point of minimum fluidisation ( U mf ) occurs when the flow velocity ( U ) is sufficiently high to support the weight of particles without transporting them out of the system [29] . U mf is defined according to the semi-empirical Ergun equation [30] : where Δ P/h is the pressure drop across a bed of height, h , ρ g is the gas density, μ g is the gas dynamic viscosity, ɛ is porosity and x p is the diameter of spherical particles. Fluidised spray granulation is a characteristically steady growth process, producing uniform well-rounded particles with a concentric layered structure [28] . We present analyses of pelletal-lapilli occurrences from southern African kimberlites that are best explained by fluidised spray granulation during emplacement. The physical properties of pelletal lapilli (e.g., uniformly coated concentric internal structure combined with a restricted particle size distribution), provide strong evidence that this process occurs when fluid, volatile-rich melts are intruded as dykes into loose, granular deposits close to the diatreme root zone. This type of multi-stage intrusion will result in spatial and temporal variation in the structure and composition of pipe-fill and consequently, could influence local diamond grade and size distributions. Venetia K1 diatreme Pelletal lapilli occur prominently in two of the world's largest diamond mines, Venetia (South Africa) and Letšeng-la-Terae (Lesotho), both well-exposed, extensively surveyed [11] , [31] , [32] and economically significant localities. The Venetia K1 diatreme was emplaced during the late-Cambrian Period (c. 519±6 Ma) [33] into metamorphic rocks of the neo-Archaean to Proterozoic Limpopo Mobile Belt (3.3–2.0 Ga). The diatreme ( Fig. 1a ) is dominated by massive volcaniclastic kimberlite (MVK; previously termed tuffisitic kimberlite breccia) [12] , a characteristically well-mixed lithofacies comprising serpentinised olivine crystals and a polymict range of lithic clasts [32] , [34] . The formation of MVK has been attributed to fluidisation [1] , [8] , [11] , the scale and context of which is heavily debated [34] , [35] . Pelletal lapilli ( Fig. 2a,b ) are confined to a narrow (10–15 m diameter), discordant and lenticular body near the northern margin of K1 ( Fig. 1a ). Although pipe-like, we refer to these features as pyroclastic intrusions to avoid confusion with the large-scale (0.5–1 km diameter) pipes or diatremes in which they occur. Field and drill-core data suggest that the intrusion is a steep-sided tapering cone, associated with numerous late phlogopite-rich dykes. The intrusion is characteristically structureless, clast- to matrix-supported, and poorly to moderately sorted. It contains abundant (90 vol%) coated lapilli-sized and very rare bomb-sized clasts ( Fig. 2a,b ), ranging in diameter from 0.2 to 100 mm (mean, =9.4 mm; Fig. 3a ). These pelletal lapilli comprise a sub-angular lithic clast or olivine macrocryst as their core surrounded by a variably thick coating (generally <1 cm); typically, this coating comprises olivine–phlogopite–spinel-bearing kimberlite with a heavily altered groundmass containing amorphous serpentine and talc. A concentric alignment of crystals is commonly developed in the coating around the core ( Fig. 2b ). In some cases, the pelletal coatings appear to have partially coalesced. 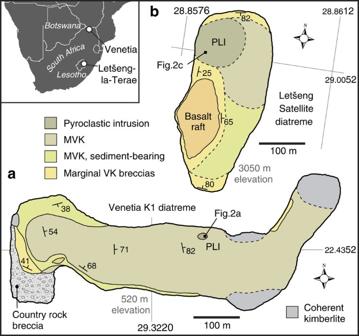Figure 1: Simplified geological maps of the Venetia and Letšeng kimberlite pipes. (a) Venetia K1 is dominated by massive volcaniclastic kimberlite (MVK, see text for details) with subordinate marginal breccias, sediment-bearing volcaniclastic kimberlite and coherent kimberlite lithofacies. The approximately 15-m-wide pelletal-lapilli intrusion (PLI) occurs near the north-central margin of the pipe, where it cross-cuts MVK and is closely associated with numerous minor late-stage dykes. (b) The Letšeng Satellite pipe is also dominated by MVK; pelletal lapilli are confined to a northern circular pipe approximately 100 m wide (modified after Palmeret al.36). Inset depicts location of the deposits in southern Africa. Figure 1: Simplified geological maps of the Venetia and Letšeng kimberlite pipes. ( a ) Venetia K1 is dominated by massive volcaniclastic kimberlite (MVK, see text for details) with subordinate marginal breccias, sediment-bearing volcaniclastic kimberlite and coherent kimberlite lithofacies. The approximately 15-m-wide pelletal-lapilli intrusion (PLI) occurs near the north-central margin of the pipe, where it cross-cuts MVK and is closely associated with numerous minor late-stage dykes. ( b ) The Letšeng Satellite pipe is also dominated by MVK; pelletal lapilli are confined to a northern circular pipe approximately 100 m wide (modified after Palmer et al . [36] ). Inset depicts location of the deposits in southern Africa. 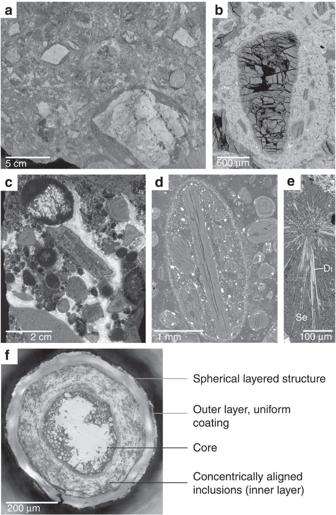Figure 2: Photographs of pelletal lapilli from southern African kimberlites and a synthetic analogue. (a) Exposure from the Venetia K1 pyroclastic intrusion showing concentrations of pelletal lapilli, which are characteristically well rounded. (b) Scanning electron microscope (SEM; backscattered-electron) image of a pelletal lapillus from (a), comprising a serpentinised olivine core and fine-grained rim comprising talc, spinel and numerous concentrically aligned micro-phenocrysts. (c) Hand specimen from Letšeng showing circular-elliptical pelletal lapilli and crystals. (d) SEM image of an elliptical pelletal lapillus from (c); note the incorporation of smaller crystals into the rim. (e) SEM image of the matrix of (d) showing the inter-growth of void-filling serpentine (Se) and diopside (Di), an assemblage indicative of low-temperature hydrothermal alteration31. (f) For comparison, a synthetic pharmaceutical granule produced by several stages of fluidised granulation; crystalline sugar core surrounded by layers of glucose, talc, polymers and cellulose (after Jacobet al.38). Full size image Figure 2: Photographs of pelletal lapilli from southern African kimberlites and a synthetic analogue. ( a ) Exposure from the Venetia K1 pyroclastic intrusion showing concentrations of pelletal lapilli, which are characteristically well rounded. ( b ) Scanning electron microscope (SEM; backscattered-electron) image of a pelletal lapillus from ( a ), comprising a serpentinised olivine core and fine-grained rim comprising talc, spinel and numerous concentrically aligned micro-phenocrysts. ( c ) Hand specimen from Letšeng showing circular-elliptical pelletal lapilli and crystals. ( d ) SEM image of an elliptical pelletal lapillus from ( c ); note the incorporation of smaller crystals into the rim. ( e ) SEM image of the matrix of ( d ) showing the inter-growth of void-filling serpentine (Se) and diopside (Di), an assemblage indicative of low-temperature hydrothermal alteration [31] . ( f ) For comparison, a synthetic pharmaceutical granule produced by several stages of fluidised granulation; crystalline sugar core surrounded by layers of glucose, talc, polymers and cellulose (after Jacob et al . [38] ). 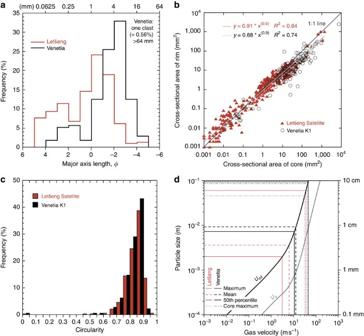Figure 3: Physical properties of pelletal lapilli from Letšeng and Venetia. (a) Step plot showing the frequency (%) of lapilli versus lapilli size in phi (φ) scale, whereφ= −Log2d, and d is the lapillus long-axis in millimetres. (b) The area of the rim is plotted against the area of the core for pelletal lapilli from both intrusions. (c) Histograms showing circularity for pelletal lapilli distributions from Letšeng and Venetia (see methods). (d) Variation in the minimum fluidisation velocity (Umf, equation (1)) and escape velocity (Ue)40for crystals and lithic clasts, fluidised by CO2at 1,000 °C (modified after Sparkset al.1). Parameter values areρs=3,300 kg m−3, to represent olivine crystals and dense lithic clasts; voidage,ɛmf=0.5 and viscosity,μ=4.62×10−6Pa s. The graph shows the gas velocities required to reachUmfandUefor a range of characteristic particle sizes (shown) for Letšeng and Venetia. Note thatUmfof the maximum lapilli size≃Ueof the mean lapilli size. The window betweenUmfandUeshows that a range of particle sizes can be supported (i.e., fluidised), but not ejected. Full size image Figure 3: Physical properties of pelletal lapilli from Letšeng and Venetia. ( a ) Step plot showing the frequency (%) of lapilli versus lapilli size in phi ( φ ) scale, where φ = −Log 2 d, and d is the lapillus long-axis in millimetres. ( b ) The area of the rim is plotted against the area of the core for pelletal lapilli from both intrusions. ( c ) Histograms showing circularity for pelletal lapilli distributions from Letšeng and Venetia (see methods). ( d ) Variation in the minimum fluidisation velocity ( U mf , equation (1)) and escape velocity ( U e ) [40] for crystals and lithic clasts, fluidised by CO 2 at 1,000 °C (modified after Sparks et al . [1] ). Parameter values are ρ s=3,300 kg m −3 , to represent olivine crystals and dense lithic clasts; voidage, ɛ mf =0.5 and viscosity, μ =4.62×10 −6 Pa s. The graph shows the gas velocities required to reach U mf and U e for a range of characteristic particle sizes (shown) for Letšeng and Venetia. Note that U mf of the maximum lapilli size ≃ U e of the mean lapilli size. The window between U mf and U e shows that a range of particle sizes can be supported (i.e., fluidised), but not ejected. Full size image Letšeng-la-Terae Satellite Pipe The Letšeng-la-Terae Satellite Pipe erupted during the Late Cretaceous Period (c.91 Ma [11] , [36] ) through Lower Jurassic flood basalts of the Drakensberg Group. Pelletal lapilli occur within a steep-sided ( ∼ 80°), 100-m-wide circular intrusion. This cross cuts MVK and marginal inward-dipping volcaniclastic breccias ( Fig. 1b ) [36] , defining a nested geometry [32] . Pelletal lapilli are characteristically well rounded ( Fig. 2c,d ), ranging in size from 60 to 61 mm ( =3.5 mm; Fig. 3a ). Pelletal cores typically constitute mantle [36] and crustal xenoliths, the most abundant being basaltic lithic clasts (85%) of presumed Drakensberg origin [11] . The rims to serpentinised olivines ( Fig. 2d ) typically consist of euhedral to subhedral olivine phenocrysts, very fine-grained chrome spinel, perovskite and titanite. The pore space is infilled by a secondary serpentine-diopside assemblage ( Fig. 2e ), which further from olivine clusters gives way to calcite [11] . The characteristics of observed pelletal lapilli ( Figs 2 and 3 ) are indicative of fluidised spray granulation [27] , [28] . This process generates well-rounded composite particles [28] , uniformly coated [37] with layered concentrically aligned inclusions ( Fig. 2f ) [38] . For both deposits, data show a moderate to strong positive correlation between the cross-sectional area of the seed particle and that of the coating ( Fig. 3b ), suggesting a uniform coating process and underlying scale invariance. Particle growth rate generally increases with increasing particle diameter [27] , because of their greater surface area. However, in this instance, larger clasts have proportionally less rim material (gradient <1; Fig. 3b ). Larger clasts have higher inertia, requiring higher sustained velocities for fluidisation, and experiencing increased abrasion at lower velocities ( U < U mf ). The circular-elliptical geometry exhibited by pelletal lapilli ( Figs 2 and 3c ) suggests their formation is governed by surface tension [1] , a major variable in fluidised spray granulation [37] . The presence of multiple rims and concentrically aligned phenocrysts in some pelletal lapilli ( Fig. 2b ) [14] is suggestive of a systematic multi-stage layering process [28] . Another key characteristic of spray granulation is the generation of a narrow particle size distribution [26] , partly due to the agglomeration of fines [26] , [27] . This is evidenced by the incorporation of small discrete rimmed crystals within larger pelletal rims ( Fig. 2b,d ). Although the Venetia and Letšeng size distributions are not strictly narrow ( Fig. 3a ), the host and proposed source material (i.e., MVK, see Fig. 1 ) has a remarkably wide size distribution, with observed crystal and lithic inclusions ranging from 0.015 to approximately 800 mm (6 to −9.7 φ ) [32] , [34] . Venetia MVK contains a high proportion of small olivine crystals (mode ≃ 0.2 mm) with proportionally fewer larger lithic clasts (mode ≃ 23 mm) resulting in a bimodal joint size distribution (Fig.6 in Walters et al . [32] ). Lapilli sizes at Letšeng and Venetia also show slight bimodality ( Fig. 3a ), but the size range is more restricted (0.03–32 mm; 5 to −5 φ ), with a higher proportion of larger lapilli (Venetia mode=5.7 mm) and a relative paucity of fine-grained particles (<0.5 mm; Fig. 3a ). To fluidise and coat the largest observed pelletal lapilli in the intrusions, gas velocities must have reached ∼ 45 m s −1 ( Fig. 3d ), broadly consistent with other estimates for MVK [1] , [32] , [34] . We emphasise, however, that the local velocity due to gas bubbles and jets is normally several times greater than the characteristic velocity of the bed [29] , [39] . Additionally, the tapered geometry gives rise to a circulating fluidised system [29] , enabling a wide range of pelletal lapilli sizes to coexist in equilibrium. For Venetia, U mf of the maximum-size lapilli is approximately equal to the escape velocity U e (the velocity at which particles escape from the system) [40] of the median-size lapilli ( Fig. 3d ). This implies there must be significant local variation in gas velocity to sustain fluidisation across the range of particle sizes observed, although retaining the smaller size fraction. For Letšeng, median particle size is considerably lower (approximately 2 mm, U mf =3 m s −1 ), suggesting greater variation in gas velocity, which can be explained by the wider vent diameter and more pronounced tapering. Clasts too large to become fluidised will behave as dispersed objects [34] . Given the high volatile contents required to generate melts of kimberlite composition (5–10 wt%) [41] , [42] , we argue that gas flow rates required to fluidise the clasts are easily achievable during degassing of a kimberlite magma. Assuming a pyroclastic intrusion diameter of 10 m, and taking gas velocities of 12 m s −1 (for the mean of the Venetia distribution; see Fig. 3d ) and 45 m s −1 (for the maximum size; see Fig. 3d ), we would require gas flow rates on the order of 942–3.5×10 3 m 3 s −1 , respectively. Our previous calculations [34] show that degassing in kimberlite root zones could result in gas mass flow rates as high as 3×10 6 m 3 s −1 , so the above estimates seem conservative. Given these estimates, a hypothetical kimberlite dyke segment of conservative length, h =10 km, breadth, b =50 m and width, 2w =2 m, containing 10% volatiles, could release sufficient gas volumes to fluidise the entire intrusion fill for tens of seconds to several minutes. As such, a degassing dyke could sustain a gas jet for long enough to efficiently entrain a significant amount of recycled pyroclasts. These results are not surprising, as comparable basaltic systems (e.g., persistently active volcanoes) can release large volumes of gas with broadly equivalent mass fluxes over significant periods of time [43] , without necessarily erupting any significant volume of degassed lava [44] . We propose that fluidised spray granulation occurs when a new pulse of kimberlite magma intrudes into unconsolidated pyroclastic deposits within the diatreme ( Fig. 4a ). The magma is transported through a dyke or system of dykes in the deep-feeding system, which at low-to-intermediate levels drive explosive volcanic flows [45] within the tapered pyroclastic intrusion. At the interface between the dyke and conduit, intensive volatile exsolution results in the formation of a gas jet [39] , where velocities are sufficiently high (order of tens of metres per second) [1] , [34] to fluidise the majority of particles ( Fig. 3d ) and inhibit formation of liquid bridges between clasts [28] . Particles from MVK are entrained into the jet because of the drag force exerted by the fluidising gas ( Fig. 4a ) [27] . Degassing is accompanied by a continuous spray of low-viscosity melt into the gas jet region [27] . Melt droplets are provided by fragmentation—the catastrophic bursting of bubbles to form a gassy spray [46] . The fragmentation level ( Fig. 4a ) will vary depending on the tensile strength of the magma [46] , which will be influenced by the ambient pressure–temperature conditions, magma rheology [47] and magma water content [1] , [46] . As melt droplets are deposited on the hot particles, they produce a thin film governed by surface tension, which dries rapidly to form a solid uniform coating [27] ( Fig. 4a,b ). Most of the very fine ash (<500 μm) is either agglomerated to the pelletal coatings [26] , [27] , [28] or elutriated by powerful gas flows [1] , [31] . Because of a combination of cohesion, high gas velocities and high fluid pressures, a fracture develops and the fluidised dispersion ascends turbulently through the diatreme fill with limited attrition and breakage ( Fig. 4b ). Fluidisation may be promoted by a sudden drop in pressure and corresponding increase in gas exsolution accompanying fracture development [48] . The lack of segregation of large lithic clasts indicates a relatively rapid termination of gas supply [34] . 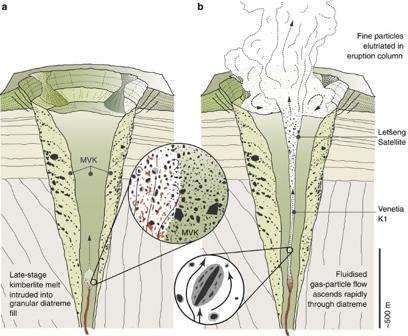Figure 4: Schematic showing the formation of pelletal lapilli in kimberlite diatremes. (a) A fluid, volatile-rich melt is intruded into loose diatreme fill; intensive volatile exsolution produces a gas-jet, opening up a fracture within MVK deposits; inset: particles from MVK are entrained and fluidised in the gas jet and uniformly coated by a spray of melt (red); fine particles are either agglomerated to pelletal coatings or elutriated by strong gas flows. (b) Driven by gas expansion and exsolution in the jet region, gas-particle dispersion ascends rapidly (>20 m s−1) and turbulently through the diatreme, and the eruption is abruptly ended. Figure 4: Schematic showing the formation of pelletal lapilli in kimberlite diatremes. ( a ) A fluid, volatile-rich melt is intruded into loose diatreme fill; intensive volatile exsolution produces a gas-jet, opening up a fracture within MVK deposits; inset: particles from MVK are entrained and fluidised in the gas jet and uniformly coated by a spray of melt (red); fine particles are either agglomerated to pelletal coatings or elutriated by strong gas flows. ( b ) Driven by gas expansion and exsolution in the jet region, gas-particle dispersion ascends rapidly (>20 m s −1 ) and turbulently through the diatreme, and the eruption is abruptly ended. Full size image Our observations from Venetia and Letšeng can be explained by dyke intrusion resulting in explosive flow processes within a narrow conduit. However, we recognise that this model will not explain all occurrences of pelletal lapilli globally, and that other important granule-forming processes may operate during eruptions. An example might include the Hawaiian-style lava fountains at the surface, where it is common for melt and gas phases to coincide with crystals and entrained clasts [49] . It is not difficult to conceive situations in which such particles could be fully supported by the viscous drag of escaping volatiles, and simultaneously, coated by a spray of fragmented low-viscosity melt. This process would provide an opportunity for recycling of previously generated pyroclasts. However, our model (see Fig. 4 ) provides a mechanism for pelletal lapilli to form at depth in pyroclastic intrusions within the vent, consistent with field relationships observed at Venetia and Letšeng. In this model, pelletal lapilli are also expected to get erupted explosively and ejected during degassing (see Fig. 4b ), producing deposits at the surface in which pelletal lapilli are volumetrically substantial. Several mechanisms could lead to incorporation of pelletal lapilli into more typical vent-filling MVK, as observed in other pipes such as Letšeng (main pipe), Wesselton, Lemphane, Liqhobong, Kao and Premier [9] , [50] . For example, pelletal lapilli ejected at the surface will get deposited in marginal bedded regions, which are capable of subsiding to deep levels in the pipe during subsequent explosive bursts at depth [51] , [52] , [53] , [54] and gas fluidisation of the pipe-fill [34] , [55] . Such large-scale fluidisation processes are thought to promote thorough mixing of pre-existing pyroclastic material [32] , [34] (including pelletal lapilli), as the vigorously fluidised dispersion effectively erodes and entrains loose material from the marginal subsided strata in the pipe [55] . It is very likely that successive eruptive phases would disrupt and disaggregate pre-existing pyroclastic intrusions, and thereby mix assemblages of pelletal lapilli together with several phases of MVK. This model is supported by the presence of steep internal contacts in kimberlite pipe-fills, separating distinct eruptive units with variable particle-size distributions [32] , [34] . Fluidised spray granulation may also help explain the welding of pyroclasts from low-viscosity magmas [56] and complex 'transition zones' between hypabyssal and diatreme-facies kimberlites [12] , [57] , [58] . Within the Venetia K1 intrusion, occasional coalesced lapilli boundaries suggest that clasts either agglomerated during circulation, or may have remained hot and partially molten during emplacement. Although sprayed kimberlite melt is likely to solidify rapidly upon contact with lithic lapilli, high magma-supply rates may lead to sustained high temperatures and the system becoming dominantly viscous with particle sintering and agglutination [59] . This would explain observed gradations to non-welded deposits and overlaps in texture and composition with adjacent pyroclastic deposits [56] . The origin of pelletal lapilli is important for understanding how magmatic pyroclasts are transported to the surface during explosive eruptions. Observed differences in juvenile composition may signify a magma with a different mantle provenance, or one that had differentiated at depth before ascent [60] . Any resulting compositional differences may be significant in terms of diamond grade (carats per tonne), size and quality. Recognising the structurally variable nature of the pipe-fill is also important for economic forecasting. For example, the Letšeng pelletal lapilli intrusion has yielded a relatively high number of large diamonds (106–215 cts), compared with the surrounding pipe-fill [36] . Spray granulation requires a strong fluidising gas flow, so our model sheds new light on the role and magnitude of fluidisation in kimberlite volcanic systems [35] . Our constraints on gas velocity provide important new inputs into thermodynamic models of kimberlite ascent and eruption, estimates of gas budget, and possibly, even magma rheology. The ability to tightly constrain gas velocities is significant, as it enables estimation of the maximum diamond size transported in the flow. Gas fluidisation and magma-coating processes are also likely to affect the diamond surface properties. Our observations also have important implications for understanding pyroclastic processes in conduits of active volcanoes (e.g., Ol Doinyo Lengai) where episodes of ash venting (commonly attributed to fluidisation) have been related to changes in eruptive activity. In such settings, pressurised CO 2 will flow through volcaniclastic deposits in the vent and crater on its way to the surface, and is likely to fluidise some of the granular material while ejecting the finer particles. The gas source is different but gives rise to the same phenomena. Our results add support to the hypothesis that pelletal lapilli in other volcanic settings are formed within the diatreme as opposed to the eruption column [21] . Most diatremes worldwide contain minor hypabyssal intrusions that cross-cut pyroclastic lithofacies [1] , [9] . When such melts penetrate loose granular deposits in the presence of rapid gas flows, we envisage that some degree of spray granulation is inevitable. On the basis of the abundance of pelletal lapilli in volcanic deposits worldwide [1] , [9] , [10] , [13] , [14] , [15] , fluidised spray granulation is likely a fundamental, but hitherto unrecognised physical process during volcanic conduit formation. Sampling and microscopy Hand specimens containing pelletal lapilli were collected from both pyroclastic intrusions ( Fig. 1 ) and analysed petrographically using optical and scanning electron microscopy (HITACHI S-3500N). High-resolution digital photographs (scaled and oriented) were taken of polished slabs and bench exposures. Particle-size distribution analysis Particle-size distribution analysis was carried out following the technique outlined in Walters et al . [32] . Because there is naturally a size limit to observable particles at any scale, samples were analysed at several overlapping scales [32] . Individual pelletal lapilli, lithic fragments and serpentinised olivine crystals were manually identified and digitised in the Adobe Illustrator (CS4) graphics package, and the resulting bitmap images were then processed in the image-analysis software package, ImageJ (developed by the US National Institute of Health; http://rsb.info.nih.gov/ij/download.html ) following Gernon et al . [11] . This provided major and minor axis measurements, cross-sectional areas for cores and rims, and circularity values (defined as 4 π ×area/perimeter 2 ; i.e., 1.0 indicates a perfect circle). How to cite this article: Gernon, T. M. et al . The origin of pelletal lapilli in explosive kimberlite eruptions. Nat. Commun. 3:832 doi: 10.1038/ncomms1842 (2012).